Telomerase expression confers cardioprotection in the adult mouse heart after acute myocardial infarction Coronary heart disease is one of the main causes of death in the developed world, and treatment success remains modest, with high mortality rates within 1 year after myocardial infarction (MI). Thus, new therapeutic targets and effective treatments are necessary. Short telomeres are risk factors for age-associated diseases, including heart disease. Here we address the potential of telomerase ( Tert ) activation in prevention of heart failure after MI in adult mice. We use adeno-associated viruses for cardiac-specific Tert expression. We find that upon MI, hearts expressing Tert show attenuated cardiac dilation, improved ventricular function and smaller infarct scars concomitant with increased mouse survival by 17% compared with controls. Furthermore, Tert treatment results in elongated telomeres, increased numbers of Ki67 and pH3-positive cardiomyocytes and a gene expression switch towards a regeneration signature of neonatal mice. Our work suggests telomerase activation could be a therapeutic strategy to prevent heart failure after MI. Chronic heart failure is a worldwide epidemic and the most common cause of mortality and morbidity worldwide, and its prevalence continues to increase. In spite of new therapies, cardiac remodelling and subsequent heart failure remain critical issues after myocardial infarction (MI) [1] , highlighting the need of developing new therapeutic strategies. MI induces profound alterations of left ventricular architecture with scar formation, ventricular dilatation and hypertrophy of the non-infarcted (remote) myocardium [2] , [3] . Ageing is one of the main risk factors for cardiovascular disease (CVD) leading to some of the above-mentioned heart alterations [4] . In addition, there is a reduction of the heart’s regenerative capacity with age [5] . In this regard, the neonatal mouse heart can undergo complete regeneration after partial surgical resection or induced MI [6] , [7] . However, this full regenerative potential is lost after the first week of life, coincidental with changes in a gene expression signature associated with regeneration [7] . Although efficient heart regeneration has been one of the goals of cardiology for the treatment of MI and prevention of heart failure, no significant advances have been made in this regard. One of the hallmarks of molecular ageing is the progressive shortening of telomeres with increasing age [8] . Indeed, short telomeres have been proposed as an age-independent risk predictor of mortality and ageing-associated diseases [9] . Mammalian telomeres are dynamic nucleoprotein structures at the ends of chromosomes [10] , [11] that consist of long stretches of 5′- TTAGGG -3′ repeats bound by a protective six-protein complex known as shelterin [11] . A minimum length of telomeric repeats is necessary for shelterin binding and telomere protection [10] , [11] . Telomerase ( Tert , telomerase reverse transcriptase) is an enzyme capable of compensating telomere attrition through de novo addition of telomeric repeats onto chromosome ends by using an associated RNA component as replication template ( Terc , telomerase RNA component) [12] . In mice and humans, telomerase is silenced after birth, leading to progressive telomere shortening throughout lifespan [13] , [14] , [15] , [16] . When telomeres reach a critically short length, this triggers activation of a persistent DNA damage response at telomeres and the subsequent induction of cellular senescence or apoptosis. In the case of adult stem cells, critical telomere shortening impairs their ability to regenerate tissues in both mice and humans, leading to age-related pathologies [17] . Notably, longitudinal studies in birds and mice show that telomere length (TL) can determine individual longevity [13] , [18] . In the case of CVD, short telomeres have been linked to cardiac dysfunction in both mice and humans [19] , [20] , [21] . Mice with critically short telomeres owing to telomerase deficiency develop cardiomyopathy characterized by impaired cell division, enhanced cardiomyocyte death and cellular hypertrophy, which are concomitant with ventricular dilation, thinning of the wall and cardiac dysfunction [19] . Interestingly, in contrast to the presence of short telomeres, telomerase mutations in humans have not been associated with CVD, presumably owing to the fact that these patients are first diagnosed with dyskeratosis congenita, aplastic anaemia or pulmonary fibrosis due to a higher proliferative index in the correspondingly affected tissues compared with the heart [22] . Analogous to the loss of the full regeneration capacity of the heart, expression of the telomerase essential genes Terc and Tert is lost within the first week of postnatal life [23] , [24] . These facts led us to speculate that telomerase re-expression in the adult heart may aid regeneration after MI. Telomerase activation has been previously explored as a strategy to elongate telomeres and delay ageing and ageing-related diseases. In the past, we were first to demonstrate that telomerase transgenic expression was sufficient to delay ageing and extend mouse longevity by 40% when in a tumour-resistant background [25] . In the case of the heart, however, Tert transgenic expression has been shown to result in increased heart hypertrophy coincidental with increased cardiomyocyte proliferation in vivo [26] . To circumvent these potential undesired effects of constitutive telomerase expression, here we used our recently developed Tert gene therapy of adult mice, which served as a proof of principle that Tert treatment of adult mice was sufficient to delay age-related pathologies and extend mouse longevity in the absence of increased cancer [27] . Of note, although Tert overexpression has been shown to affect gene expression independently of its catalytic activity [28] , we previously demonstrated that Tert effects on delaying ageing and increasing longevity require its catalytic activity [27] ; thus, for all the experiments described here we used wild-type (WT) Tert . Here we address the potential therapeutic effects of Tert expression in MI using adeno-associated viruses of serotype 9—AAV9—in a mouse model of MI induced by coronary artery ligation. We find that Tert re-activation in the adult mouse heart improves cardiac functional and morphological parameters, induces cardio-protective pathways and significantly reduces mortality by heart failure after MI. These findings are a proof of principle that Tert treatment of the adult mouse heart has beneficial effects in improving heart function and organismal survival after MI. Tert expression is suppressed during the first week of life We first set out to determine whether mouse Tert expression is downregulated in the heart during the first week of life, similar to that previously described for mouse telomerase RNA component in different mouse tissues [23] , Terc , as well as for Tert expression in the rat [24] . To this end, we isolated neonatal hearts at days 1, 3, 7 and 10, and determined mouse Tert expression by quantitative reverse transcriptase–PCR (qRT–PCR). We observed a significant dowregulation of mouse Tert messenger RNA levels from day 7 after birth ( Supplementary Fig. 1 ). Targeting AAV9- Tert specifically to the heart Next, we set to deliver mouse Tert expression specifically to the adult heart. AAV9 is known to preferentially target the heart and the liver when administered systemically, although the efficiency of targeting hepatocytes is around tenfold lower than that of targeting cardiomyocytes [29] . We used this differential transduction efficiency to find a minimal dose of AAV9 vectors that would specifically target the heart, with minimal transduction of the liver, and other tissues. Under our experimental conditions, a dose 5 × 10 11 vg per mouse of a AAV9 reporter vector (AAV9-CMV-eGFP) could transduce >60% of heart cells, as shown by enhanced green fluorescent protein (eGFP) immunohistochemistry ( Fig. 1a,c ), but <1.2% of liver and brain cells ( Fig. 1b,c ). 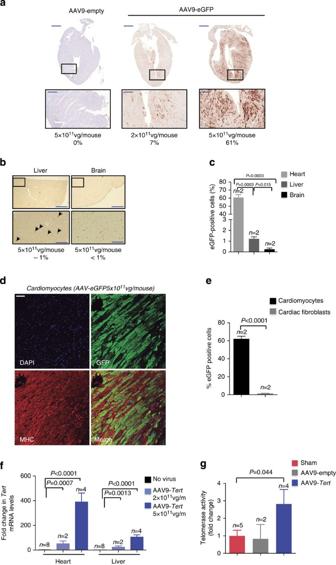Figure 1: Specific targeting ofTertto the heart. (a) Anti-eGFP immunohistochemistry to assess tropism of AAV9-eGFP viruses to the myocardium. Different concentrations of viruses are indicated. Scale bars, 1,000 μm (top row); (200 μm) in higher magnification images. (b) Tropism at the indicated AAV9-eGFP viral concentration to the liver and brain. Scale bars, 1,000 μm (top row); 200 μm (bottom row). Black arrows indicate eGFP-positive cells. (c) Percentage of viral transduction in the indicated tissues. (d) AAV9 specifically transduces cardiomyocytes. Co-immunostaining of LV tissue section was done with anti-myosin heavy chain (MHC) to stain cardiomyocytes (red) and with anti-eGFP (green) antibodies to identify infected cardiomyocytes. Cell nuclei were stained with DAPI (blue). Scale bar, 50 μm. (e) Percentage of eGFP-positive (AAV9 infected) cardiomyocytes or cardiac fibroblasts. (f) Fold changes in mRNA levels ofTertafter injection of different AAV9-Tertdoses in the heart and liver relative to non-injected animals (no virus). (g) Telomerase activity in extracts of sham and MI hearts infected with AAV9-empty or AAV9-Tertwas determined following the telomeric repeat amplification protocol (TRAP). All graphs show mean values, error bars indicate s.e.m,n=number of mice. Two-sided Student’st-test was used for statistical analysis andP-values are shown. To estimate the transduction efficiency of the telomerase vector (AAV9-CMV- Tert ; hereafter AAV9- Tert ), we compared the viral genome copy number per diploid genome in hearts transduced with either the eGFP reporter vector or the AAV9- Tert vector ( Table 1 ). We found similar numbers of viral genome copies per cell, indicating similar transduction efficiency for AAV9-eGFP and AAV9- Tert in the heart. Using co-immunostaining with eGFP and markers of either cardiomyocytes ( β -myosin heavy chain) or fibroblasts (vimentin), we found that within the myocardium, AAV9 preferentially targets cardiomyocytes (>60% eGFP-positive cardiomyocytes; Fig. 1d,e ), while we found no evidence for infection of fibroblasts ( Fig. 1e and Supplementary Fig. 2 ). Specific targeting of Tert to the heart was also confirmed by qRT–PCR showing a ~400-fold induction of Tert mRNA amounts in the heart of treated mice compared with non-treated mice, while Tert mRNA upregulation was 40-fold lower in the liver of treated mice ( Fig. 1f ). Tert mRNA expression levels in heart remained high during at least 2 months as indicated by >200-fold increased expression in AAV9- Tert -treated mice compared with those treated with the empty vector ( Supplementary Fig. 3a ). Finally, increased Tert mRNA expression was paralleled by increased TERT protein expression and increased telomerase activity in the AAV9- Tert -treated hearts compared with non-treated mice and AAV9-empty-treated controls ( Supplementary Fig. 3b,c and Fig. 1g ). Of note, on AAV9- Tert treatment the fold increase in Tert mRNA expression levels is higher than the fold increase in protein expression/telomerase activity, as previously observed by us using both classical transgenesis and the AAV9 system [25] , [27] , [30] . Together, these results indicate that we achieved specific Tert expression in the adult heart. Figure 1: Specific targeting of Tert to the heart. ( a ) Anti-eGFP immunohistochemistry to assess tropism of AAV9-eGFP viruses to the myocardium. Different concentrations of viruses are indicated. Scale bars, 1,000 μm (top row); (200 μm) in higher magnification images. ( b ) Tropism at the indicated AAV9-eGFP viral concentration to the liver and brain. Scale bars, 1,000 μm (top row); 200 μm (bottom row). Black arrows indicate eGFP-positive cells. ( c ) Percentage of viral transduction in the indicated tissues. ( d ) AAV9 specifically transduces cardiomyocytes. Co-immunostaining of LV tissue section was done with anti-myosin heavy chain (MHC) to stain cardiomyocytes (red) and with anti-eGFP (green) antibodies to identify infected cardiomyocytes. Cell nuclei were stained with DAPI (blue). Scale bar, 50 μm. ( e ) Percentage of eGFP-positive (AAV9 infected) cardiomyocytes or cardiac fibroblasts. ( f ) Fold changes in mRNA levels of Tert after injection of different AAV9- Tert doses in the heart and liver relative to non-injected animals (no virus). ( g ) Telomerase activity in extracts of sham and MI hearts infected with AAV9-empty or AAV9- Tert was determined following the telomeric repeat amplification protocol (TRAP). All graphs show mean values, error bars indicate s.e.m, n =number of mice. Two-sided Student’s t -test was used for statistical analysis and P -values are shown. Full size image Table 1 Ratio of viral genomes per diploid genome. Full size table Telomerase expression does not alter heart morphology Constitutive Tert transgenic expression in the heart from embryonic development onwards results in heart hypertrophy [26] . Thus, we first set to determine whether AAV9- Tert treatment during adulthood had any undesired effects on heart morphology. AAV9- Tert treatment in the absence of MI did not change the normal heart structure nor did produce any signs of cardiac hypertrophy as assessed 9–10 weeks after virus administration ( Supplementary Fig. 3d ). Further supporting a normal structure of the heart, we found normal expression of β -myosin heavy chain in AAV9- Tert -treated hearts ( Supplementary Fig. 3e ). These results indicate that Tert overexpression by means of AAV9 gene therapy does not have any of the adverse effects previously reported for constitutive Tert transgenic expression in the heart. In line with AAV9- Tert expression per se , having no dramatic effects in heart morphology, we compared the hearts of WT, Tert heterozygous and first generation (G1) Tert -deficient mice, and found no significant morphological changes on histopathological analysis ( Supplementary Fig. 4 ). These results are in agreement with previous data demonstrating that morphological alterations in the mouse heart start to emerge only in late generations of mice deficient for the telomerase RNA component or Terc [19] . Telomerase gene therapy reduces mortality after MI To assess the therapeutic potential of telomerase activation during adulthood in prevention of heart failure after MI, we used a bona fide mouse pre-clinical model of MI after coronary artery ligation, previously shown to recapitulate heart failure induced by MI [31] ( Supplementary Fig. 5a,b ). In particular, we used FVB/N mice, as the main cause of death in these mice after MI is lethal heart failure (as opposed to heart rupture, for example, in C57/BL6) [31] and this reflects the situation found in humans. Of note, FVB/N mice also exhibit similarly long telomeres compared with other laboratory mouse strains previously used for telomere analysis (for example, C57/Bl6) [32] , thus making the FVB/N mice optimal for our study. Cardiac-specific AAV9-mediated transgene expression reaches its maximum after around 2 weeks and remains stable thereafter [33] . Even though expression emerges already very shortly after intravenous injection, we decided to induce MI 2–3 weeks after virus administration, to assure Tert levels are maximal. Furthermore, as we were interested in regeneration and remodelling processes after acute infarction, which in humans predominantly occurs in the adult life, we used adult (1-year-old) mice. All mice under experimentation were males to avoid gender bias. Interestingly, a single treatment with AAV9- Tert 3 weeks before artery ligation was sufficient to rescue mouse survival post infarction, with >74% of the AAV9- Tert -treated mice surviving infarct compared with only 57% of those treated with the empty vector ( Fig. 2a ). Thus, telomerase activation in adult mice significantly reduces mortality by heart failure after MI in a bona fide mouse model for the human condition. 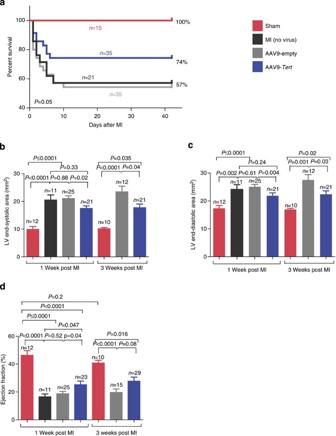Figure 2:Tertreduces mortality and rescues cardiac function after MI. (a) Kaplan–Meier survival curves after MI, indicating 17% improved survival afterTerttreatment and MI. Statistical analysis was calculated χ2-test.n, number of mice. (b–d) Echocardiography at 1 and 3 weeks in mice injected with AAV9-Tert(blue bars), AAV9-empty (light grey bars) or no virus (dark grey bars) (all three groups suffered MI); or sham-operated mice (red bars) (no virus, no MI) reveals functional improvement in theTert-treated group. Note, same colours are used throughout the paper. (b) LV end-systolic area, (c) LV end-diastolic area, (d) ejection fraction.n, number of mice; bars show mean values with s.e.m. (error bars). Two-sided Student’st-test was used for statistical analysis andP-values are shown. Figure 2: Tert reduces mortality and rescues cardiac function after MI. ( a ) Kaplan–Meier survival curves after MI, indicating 17% improved survival after Tert treatment and MI. Statistical analysis was calculated χ 2 -test. n , number of mice. ( b – d ) Echocardiography at 1 and 3 weeks in mice injected with AAV9- Tert (blue bars), AAV9-empty (light grey bars) or no virus (dark grey bars) (all three groups suffered MI); or sham-operated mice (red bars) (no virus, no MI) reveals functional improvement in the Tert -treated group. Note, same colours are used throughout the paper. ( b ) LV end-systolic area, ( c ) LV end-diastolic area, ( d ) ejection fraction. n , number of mice; bars show mean values with s.e.m. (error bars). Two-sided Student’s t -test was used for statistical analysis and P -values are shown. Full size image Telomerase gene therapy improves cardiac function after MI To investigate how telomerase expression results in lower mortality rates on MI, cardiac function was assessed by two-dimensional echocardiography [34] at 1 and 3 weeks after left anterior descending (LAD) ligation. Cardiac dimensions such as left ventricle (LV) systolic and diastolic area were strongly increased after MI compared with the sham-operated (no MI) mice ( Fig. 2b,c ), which consequently results in decreased cardiac ejection fractions ( Fig. 2d ). Importantly, the ejection fractions were significantly rescued in mice that received the Tert gene therapy but not in those that received the empty vector ( Fig. 2b ). Next, we performed positron emission tomography (PET) scan analysis using fluorodeoxyglucose (FDG) as tracer, a diagnostic tool commonly used to assess infarct severity in vivo , as it measures metabolic activity in the heart via determining glucose uptake by cardiomyocytes. In particular, heart infarct results in decreased metabolic activity at the damaged regions [35] . First, we noticed that AAV9- Tert -treated mice present a better survival to the PET procedure per se , which involves anaesthesia and may result in death of mice subjected to MI ( Fig. 3a ). Of note, survival curves shown in Fig. 2a do not include mice used for PET. As expected, all mice showed reduced PET signals indicative of MI at 4 weeks after LAD ligation; however, we observed less severe infarcts (characterized by >50% loss of the PET signal) in the AAV9- Tert -treated group compared with the AAV9-empty-treated group ( Fig. 3b,c ). These results indicate that AAV9- Tert -treated hearts show a better preservation of metabolically active regions compared with the AAV9-empty group on MI. 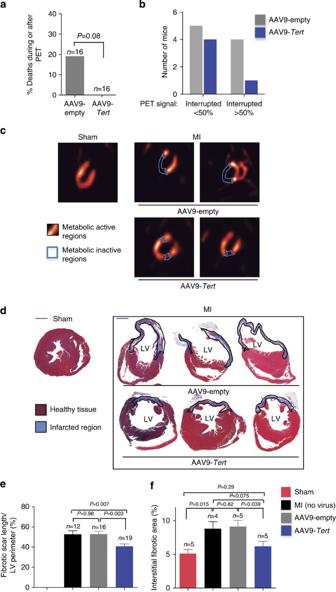Figure 3: Reduced infarct severity coincides with less fibrosis. (a) Percentage of AAV9-empty or AAV9-Tertmice that died during or shortly after PET scan.n, number of mice. Statistical analysis: χ2-test,P-value is depicted. (b) Infarct severity in AAV9-Tertand AAV9-empty cohorts was assessed inin vivoFDG-PET scans 4 weeks after LAD ligation. A higher number of hearts with signal loss was found in the AAV9-empty group. (c) Representative PET scan images of a fully functional heart (left) and failing hearts after MI (right). (d) Representative Masson’s trichrome stainings of transverse heart sections of a healthy heart (left) and LAD ligated hearts with infarct scar (right). Fibrotic infarct areas stain in blue and infarct remote in red as indicated. Scale bar, 1mm. (e) Average scar length relative to the LV endocardial circumference of indicated groups shown as mean with s.e.m. (f) Interstitial fibrotic area relative to total area measured in the infarct remote myocardium shown as mean with s.e.m.n, number of mice. Statistical analysis: two-sided Student’st-test,P-values are shown. Figure 3: Reduced infarct severity coincides with less fibrosis. ( a ) Percentage of AAV9-empty or AAV9- Tert mice that died during or shortly after PET scan. n , number of mice. Statistical analysis: χ 2 -test, P -value is depicted. ( b ) Infarct severity in AAV9- Tert and AAV9-empty cohorts was assessed in in vivo FDG-PET scans 4 weeks after LAD ligation. A higher number of hearts with signal loss was found in the AAV9-empty group. ( c ) Representative PET scan images of a fully functional heart (left) and failing hearts after MI (right). ( d ) Representative Masson’s trichrome stainings of transverse heart sections of a healthy heart (left) and LAD ligated hearts with infarct scar (right). Fibrotic infarct areas stain in blue and infarct remote in red as indicated. Scale bar, 1mm. ( e ) Average scar length relative to the LV endocardial circumference of indicated groups shown as mean with s.e.m. ( f ) Interstitial fibrotic area relative to total area measured in the infarct remote myocardium shown as mean with s.e.m. n , number of mice. Statistical analysis: two-sided Student’s t -test, P -values are shown. Full size image Six weeks after MI, we performed full pathological analysis including determination of heart scar length using Masson’s trichrome staining (blue—fibrotic infarct area; red—non-infarcted myocardium) ( Fig. 3d and Supplementary Fig. 6 ). We found that AAV9- Tert -treated mice presented smaller infarcts compared with AAV-empty or no virus controls, as determined by the ratio of scar length to endocardial circumference ( Fig. 3e ). This difference is unlikely to result from AAV9- Tert -treated mice having received smaller heart injuries, as we observed no differences in fibrotic scar size between AAV9- Tert and AAV9-empty-treated mice that died from lethal heart failure between 5 and 7 days after MI was performed ( Supplementary Fig. 7a,b ). In addition, AAV9- Tert mice developed less interstitial fibrosis in the non-infarcted region of the LV compared with the AAV9-empty group ( Fig. 3f ). Together, these findings indicate that a single AAV9- Tert treatment resulted in increased survival of the myocardium and smaller infarct sizes, thus preventing heart functional decline after MI. Telomerase treatment rescues short telomeres in the heart Critical telomere shortening causes heart dysfunction in mice. In particular, telomerase-deficient mice bearing critically short telomeres present heart phenotypes resembling those of heart dysfunction in humans, including heart hypertrophy [19] . As the main function of telomerase is to elongate critically short telomeres, here we set out to address the effects of Tert treatment on heart TL by performing quantitative fluorescent in situ hybridization (Q-FISH) of telomere lengths directly on heart sections. We found that AAV9- Tert -treated hearts show a net increase in TL and a lower abundance of cells with short telomeres (represented as 20th percentile of TL in the AAV9-empty-treated hearts) in the infarct remote area compared with the empty vector group ( Fig. 4a–c ). Thus, AAV9- Tert is a potent tool to decrease the abundance of short telomeres in the myocardium and, subsequently, the associated risk of heart failure in a short period of time (TL was measured 9–10 weeks after virus administration). These results are consistent with our previous findings that AAV9- Tert gene therapy leads to longer TL in the uninjured heart [27] . However, we do not rule out the possibility that MI itself could lead to telomere shortening, and that this would be less severe in the Tert -treated hearts. In addition to measuring TL in heart tissue, and as short telomeres in peripheral blood leukocytes in humans are a marker for cardiovascular ageing and a risk factor for CVDs, we also measured TL in the blood. We found a tendency to have longer telomeres in blood cells from AAV9- Tert -injected mice compared with the AAV9-empty controls ( Fig. 4d ), although it did not reach significance in agreement with specific targeting of Tert to the heart in this study. No differences in blood TL were observed between sham-operated mice and those that underwent MI and received AAV9-empty or no virus. These findings suggest that acute MI and the subsequent inflammation events, which are processes known to be associated with telomere shortening in blood under certain chronic conditions [36] , do not negatively have an impact on TL in the blood. 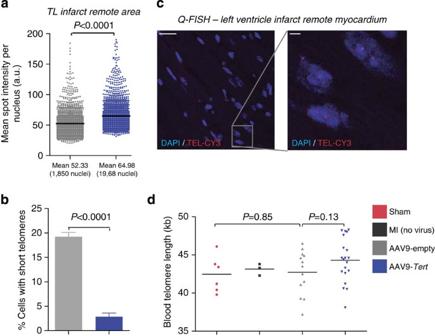Figure 4: Telomerase expression results in longer telomeres in cardiac cells. (a) TL was determined by Q-FISH analysis on heart tissue sections after MI in the left ventricular infarct remote area in mice transduced with AAV9-Tertand AAV9-empty. Four animals (hearts) per group were analysed (n=4). TL is represented as mean telomere fluorescence per nucleus in arbitrary units of fluorescence (a.u.). The black line indicates mean TL. Statistical analysis: two-sided Student’st-test,P-values are depicted. Scale bar, 25 μm. (b) Fractions of nuclei per mouse (from A), which fall below the 20th percentile of the control (AAV9-empty) TL are represented as the percentage of cells with short telomeres. Statistical analysis: two-sided Student’st-test,P-values are shown. (c) Representative images of heart sections subjected to telomere Q-FISH analysis. Nuclei are stained with DAPI and telomeres with a specific CY3-labelled probe. Nuclei stained with DAPI (blue) and telomeres with CY3-labelled probe (red). Scale bars, 20 μm (left image); 2 μm (zoom in). (d) TL (in kb) measured in peripheral blood leukocytes by using HT-Q-FISH technology. Each spot represents the mean TL of one individual mouse (from left to rightn=6, 3, 13, 20). Mean TL among all mice per group is indicated by the black horizontal lines. Statistical analysis: two-sided Student’st-test,P-values are shown. Figure 4: Telomerase expression results in longer telomeres in cardiac cells. ( a ) TL was determined by Q-FISH analysis on heart tissue sections after MI in the left ventricular infarct remote area in mice transduced with AAV9- Tert and AAV9-empty. Four animals (hearts) per group were analysed ( n =4). TL is represented as mean telomere fluorescence per nucleus in arbitrary units of fluorescence (a.u.). The black line indicates mean TL. Statistical analysis: two-sided Student’s t -test, P -values are depicted. Scale bar, 25 μm. ( b ) Fractions of nuclei per mouse (from A), which fall below the 20th percentile of the control (AAV9-empty) TL are represented as the percentage of cells with short telomeres. Statistical analysis: two-sided Student’s t -test, P -values are shown. ( c ) Representative images of heart sections subjected to telomere Q-FISH analysis. Nuclei are stained with DAPI and telomeres with a specific CY3-labelled probe. Nuclei stained with DAPI (blue) and telomeres with CY3-labelled probe (red). Scale bars, 20 μm (left image); 2 μm (zoom in). ( d ) TL (in kb) measured in peripheral blood leukocytes by using HT-Q-FISH technology. Each spot represents the mean TL of one individual mouse (from left to right n =6, 3, 13, 20). Mean TL among all mice per group is indicated by the black horizontal lines. Statistical analysis: two-sided Student’s t -test, P -values are shown. Full size image Tert treatment does not enhance hypertrophy after MI To test whether Tert treatment induces a stronger hypertrophic response to cardiac damage, we performed morphometric analysis of histological heart sections from mice that received MI 6 weeks before analysis ( Supplementary Fig. 8a,b ). We do not find evidence supporting an increased hypertrophic response as indicated by similar LV mass ( Supplementary Fig. 8c ), LV mass index ( Supplementary Fig. 8d ) and cardiomyocyte cross-sectional area ( Supplementary Fig. 8e in mice treated with AAV9-empty or AAV9- Tert , which is in agreement with undetectable morphological changes in sham-operated animals ( Supplementary Fig. 3d ). Tert increases number of cycling cardiomyocytes To study the impact of Tert treatment on apoptosis and proliferation in the heart after MI, we quantified the percentage of cells showing active caspase-3 and Ki67-positive staining, respectively, 6 weeks post MI. We found very few apoptotic cells 6 weeks post MI regardless of the treatment ( Supplementary Fig. 9a,b ), in agreement with the fact that apoptosis is an early response following ischaemia [37] . On MI, we observed increased cycling Ki67-positive cells in the infarct remote area and in the infarct area both in the AAV9- Tert and the AAV9-empty groups compared with the sham-operated mice ( Supplementary Fig. 10a ). However, this increase was significantly attenuated in the AAV9- Tert group compared with AAV9-empty ( Supplementary Fig. 10b ), in line with decreased fibrotic scar formation in these mice. Interestingly, co-immunostaining using Ki67 and the cardiomyocyte marker Troponin T ( Fig. 5a ) and MHC ( Supplementary Fig. 11a ) showed the presence of Ki67-positive cardiomyocytes in the infarct vicinity reaching ~0.2% of the total cells in the AAV9-empty-treated hearts, which is similar to that described in previous studies [19] , [38] . This number was significantly increased to ~0.5% in the AAV9- Tert -treated group ( Fig. 5b ). To further characterize cycling cardiomyocytes, we acquired Z -stacks and performed three-dimensional reconstructions, which confirmed that the Ki67 nuclei belong to cardiomyocytes ( Supplementary Fig. 11b,c ). To test whether cardiac cells also enter mitosis, we performed immunostaining using the phospho-histon 3 marker (pH3). Consistent with pH3 being expressed only in M-phase of the cell cycle in contrast to Ki67 that is expressed in G1, M, G2 and S-phases [39] , we found lower numbers of pH3-positive cells compared with Ki67-positive cells ( Fig. 5c ). Interestingly, we found a threefold increase in anti-pH3-labelled cardiomyocytes in Tert -treated hearts compared with the empty virus group ( Fig. 5d ). 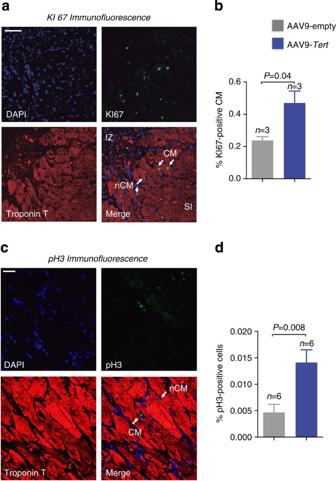Figure 5:Tertleads to an increase in Ki67- and pH3-positive cardiomyocytes. (a) Representative confocal immunofluorescence images demonstrating co-localization of Ki67 (green) and the cardiomyocyte marker Troponin T (red) in the infarct vicinity. Nuclei stained in blue with DAPI. (IZ, infarct zone; SI, subinfarct zone; CM, cardiomyocyte; nCM, non-cardiomyocyte). Scale bar, 50 μm. (b) Quantification of Ki67-positive cardiomyocytes in the infarct adjacent area given as percentage of total cells. Four to eight fields of three mice each per group were counted (n=3). (c) Representative confocal immunofluorescence images demonstrating co-localization of pH3 (green) and the cardiomyocyte marker Troponin T (red) in the infarct vicinity (CM, cardiomyocyte; nCM, non-cardiomyocyte). DAPI-stained nuclei in blue. Scale bar, 25 μm. (d) Quantification of pH3-positive cardiomyocytes in the infarct adjacent area given as percentage of total cells. Thirty fields per heart and six mice of each group were counted (n=6). Bar graphs show mean values with s.e.m. Statistical analysis: two-sided Student’st-test,P-values are shown. Figure 5: Tert leads to an increase in Ki67- and pH3-positive cardiomyocytes. ( a ) Representative confocal immunofluorescence images demonstrating co-localization of Ki67 (green) and the cardiomyocyte marker Troponin T (red) in the infarct vicinity. Nuclei stained in blue with DAPI. (IZ, infarct zone; SI, subinfarct zone; CM, cardiomyocyte; nCM, non-cardiomyocyte). Scale bar, 50 μm. ( b ) Quantification of Ki67-positive cardiomyocytes in the infarct adjacent area given as percentage of total cells. Four to eight fields of three mice each per group were counted ( n =3). ( c ) Representative confocal immunofluorescence images demonstrating co-localization of pH3 (green) and the cardiomyocyte marker Troponin T (red) in the infarct vicinity (CM, cardiomyocyte; nCM, non-cardiomyocyte). DAPI-stained nuclei in blue. Scale bar, 25 μm. ( d ) Quantification of pH3-positive cardiomyocytes in the infarct adjacent area given as percentage of total cells. Thirty fields per heart and six mice of each group were counted ( n =6). Bar graphs show mean values with s.e.m. Statistical analysis: two-sided Student’s t -test, P -values are shown. Full size image Impacts on metabolic and signalling networks related to MI To further understand the role of Tert in protection from acute heart failure after MI, we first studied changes in serum metabolites in the different mouse cohorts. Owing to a drastically lowered ejection fraction ( Fig. 2d ), MI can reduce the blood flow to the kidney and eventually induce kidney dysfunction with reduced glomerular filtration rates leading to increased urea blood levels. We found that 6 weeks after MI, serum urea levels were significantly increased in mice treated with no virus or with the empty vector, and that this was significantly rescued in the AAV9- Tert cohort ( Fig. 6a ). A better renal function on MI in AAV9- Tert -treated mice supports our findings of improved cardiac function in these mice ( Fig. 2b–d ). 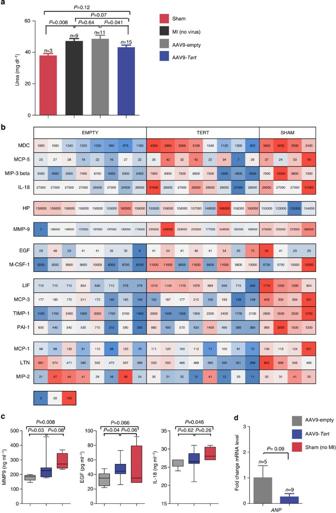Figure 6:Tertrescues serum parameters associated with heart failure. (a) Serum urea concentration as a measure of renal and heart functionality was determined in the indicated groups.n, number of mice. Statistical analysis: two-sided Student’st-test,P-values are shown. (b) Individual heatmaps (from blue—lowest, to red—highest value) of serum concentration of the indicated biomarkers comparing three conditions: MI+AAV9-empty (n=8), MI+AAV9-Tert (n=8), sham (no virus) (n=4).n, number of mice. The indicated numbers within squares represent true values in pg μl−1serum. (c) A selection of serum biomarkers with implications in heart biology that show significant changes between MI and sham animals as determined in multi-analyte profiling represented as box and whiskers plot. Statistical analysis: Mann–WhitneyU-test,P-values are shown. (d) Relative mRNA expression level (qRT–PCR) ofANPin non-infarcted mice (>2years). Mean values with s.e.m are represented.n, number of mice. Statistical analysis: two-sided Student’st-test,P-values are shown. Figure 6: Tert rescues serum parameters associated with heart failure. ( a ) Serum urea concentration as a measure of renal and heart functionality was determined in the indicated groups. n , number of mice. Statistical analysis: two-sided Student’s t -test, P -values are shown. ( b ) Individual heatmaps (from blue—lowest, to red—highest value) of serum concentration of the indicated biomarkers comparing three conditions: MI+AAV9-empty ( n =8), MI+AAV9-Tert ( n =8), sham (no virus) ( n =4). n , number of mice. The indicated numbers within squares represent true values in pg μl −1 serum. ( c ) A selection of serum biomarkers with implications in heart biology that show significant changes between MI and sham animals as determined in multi-analyte profiling represented as box and whiskers plot. Statistical analysis: Mann–Whitney U -test, P -values are shown. ( d ) Relative mRNA expression level (qRT–PCR) of ANP in non-infarcted mice (>2years). Mean values with s.e.m are represented. n , number of mice. Statistical analysis: two-sided Student’s t -test, P -values are shown. Full size image Next, we performed a comprehensive serum multi-analyte profiling 6 weeks post MI encompassing various biological pathways ( Supplementary Table 1 ; biomarkers below detection limit or with flat profile (no changes between groups) are indicated). We found that MI resulted in significant decrease in the serum levels of factors involved in tissue remodelling such as metalloproteinases (matrix metalloproteinase-9) and their inhibitors (tissue inhibitors of metalloproteinase-1 (TIMP-1)) [40] , in inflammation such as MDC (macrophage-derived chemokine) or interleukin 18, and in the epidermal growth factor (EGF) ( Fig. 6b,c ). Importantly, all of them were partially rescued in the AAV9- Tert group ( Fig. 6b,c ). Of interest, increased EGF receptor has been previously described as cardio protective [41] . Next, we determined the expression of the atrial natriuretic peptide (ANP), a fetal heart protein, which is repressed after birth together with other fetal heart genes, but greatly increases during late stages of heart failure [2] . Interestingly, ANP levels were decreased following AAV9- Tert treatment in old WT hearts (non-infarcted >2 years old mice) ( Fig. 6d ), suggesting that Tert treatment represses the pathological expression of fetal genes. To gain further insights into the gene expression changes mediated by Tert in the heart, we performed microarray DNA analysis 6 weeks post MI, which reflect later stages of tissue repair process, including cardiac remodelling and scar formation [37] . We used RNA from left ventricular heart tissue from the different groups (sham (no MI); MI+AAV9- Tert ; MI+AAV9-empty). Gene set enrichment analysis (GSEA) revealed upregulation of pathways associated with inflammation, proliferation and DNA replication in the infarcted mice compared with the sham group (no MI) ( Fig. 7a and Supplementary Table 3 ), which were significantly rescued in AAV9- Tert -treated mice compared with AAV9-empty controls ( Fig. 7a and Supplementary Table 2 ). Relative overexpression of repair pathways in AAV9-empty can readily be explained by a stronger repair response and increased proliferation of fibroblasts [42] (that is, fibrotic damage repair) and can be seen by a relative abundance of pathways associated with DNA repair/replication (for example, ‘activation of Atr in response to replicative stress’). Consistent with enforced Tert overexpression, we find significant differential expression in the gene set termed ‘extension of telomeres’. Moreover, increased inflammation is attributed to the clearance of apoptotic and necrotic cardiomyocytes on MI. Thus, the fact that Tert attenuates the expression of genes involved in inflammation and proliferation supports our functional findings that AAV9- Tert treatment is cardio protective. Moreover, we found a significant enrichment in several signatures related to remodelling of the extracellular matrix and fibroblasts dynamics (for example, extracellular matrix (ECM), transforming growth factor-β (TGF-β) and fibroblast growth factor receptor) in the Tert -treated group compared with the empty vector controls ( Fig. 7b ). We confirmed some of the most differentially expressed genes within these gene sets ( Fgfr3 and Bmpr1b , respectively) by qRT–PCR ( Fig. 6c ). In addition, Timp1 , Thbs1 and Thbs4 (thrombospondin 1 and 4) were also differentially expressed in Tert -treated mice ( Supplementary Table 2 ). Increased Timp1 expression is in agreement with higher TIMP-1 protein levels in the serum from Tert -treated mice ( Fig. 6e ). These findings are of interest given that overexpression of Timp 1 has been shown to mitigate adverse myocardial remodelling and to improve cardiac function, while Thbs1 and Thbs4 are important regulators of cardiac adaptation post MI by regulating fibrosis and remodelling of the myocardium [43] , [44] , [45] . 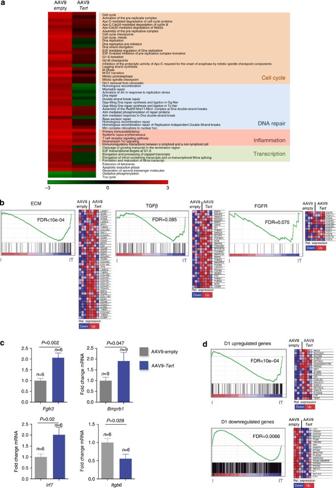Figure 7: Gene expression changes induced byTertexpression in the heart. (a) Summary table indicating that various gene sets are differentially regulated in the comparisons MI versus sham andTert(MI) versus empty (MI). The corresponding affected biological pathways are indicated. (b) GSEA plots for the indicated pathways in heart tissue. Microarray genes were ranked based on the two-tailedt-statistic tests obtained from the AAV9-Tertversus AAV9-empty by pair-wise comparisons. The red to blue horizontal bar represents the ranked list. Those genes showing higher expression levels for each cohort are located at the edges of the bar (I=infarct+AAV9-empty; IT infarct+AAV9-Tert). The genes located at the central area of the bar show small differences in gene expression fold changes between both groups. A heatmap of indicated core-enriched genes is displayed on the right of each enrichment plot. (c) Relative mRNA expression level (qRT–PCR) ofFgfr3,Bmpr1b,Irf7andItgb6in AAV9-empty versus AAV9-Tertconfirm candidate genes found among the most differentially expressed genes in GSEA represented as fold change relative to AAV9-empty group.n, number of mice. Mean values with s.e.m are represented. Statistical analysis: two-sided Student’st-test,P-values are shown. (d) GSEA analysis reveals a regenerative signature inTert-treated mice. The represented gene sets were generated using the expression profiles in neonatal mice (day1=D1) described by Haubneret al.7Selections for up- and downregulated genes were based on FDR values <0.01 in their comparison of gene expression profiles between D1 and D10. For GSEA Kolmogorov–Smirnoff testing was used for statistical analysis. The FDR is calculated by Benjamini and Hochberg FDR correction. Figure 7: Gene expression changes induced by Tert expression in the heart. ( a ) Summary table indicating that various gene sets are differentially regulated in the comparisons MI versus sham and Tert (MI) versus empty (MI). The corresponding affected biological pathways are indicated. ( b ) GSEA plots for the indicated pathways in heart tissue. Microarray genes were ranked based on the two-tailed t -statistic tests obtained from the AAV9- Tert versus AAV9-empty by pair-wise comparisons. The red to blue horizontal bar represents the ranked list. Those genes showing higher expression levels for each cohort are located at the edges of the bar (I=infarct+AAV9-empty; IT infarct+AAV9- Tert ). The genes located at the central area of the bar show small differences in gene expression fold changes between both groups. A heatmap of indicated core-enriched genes is displayed on the right of each enrichment plot. ( c ) Relative mRNA expression level (qRT–PCR) of Fgfr3 , Bmpr1b , Irf7 and Itgb6 in AAV9-empty versus AAV9- Tert confirm candidate genes found among the most differentially expressed genes in GSEA represented as fold change relative to AAV9-empty group. n , number of mice. Mean values with s.e.m are represented. Statistical analysis: two-sided Student’s t -test, P -values are shown. ( d ) GSEA analysis reveals a regenerative signature in Tert -treated mice. The represented gene sets were generated using the expression profiles in neonatal mice (day1=D1) described by Haubner et al . [7] Selections for up- and downregulated genes were based on FDR values <0.01 in their comparison of gene expression profiles between D1 and D10. For GSEA Kolmogorov–Smirnoff testing was used for statistical analysis. The FDR is calculated by Benjamini and Hochberg FDR correction. Full size image Neonatal mice have full regenerative potential during the first week of life, which is characterized by a highly proliferative state of cardiomyocytes and a well-defined gene expression signature [7] . Thus, we next set out to address whether gene expression changes associated with Tert treatment in adult hearts were enriched in the regenerative gene expression signature described in neonatal mice. Strikingly, by comparing our expression data with genes overexpressed or underrepresented at postnatal day 1 (relative to postnatal day 10) [7] , a stage at which the heart possesses full regenerative potential after MI, we found a significant enrichment in the AAV9- Tert group compared with AAV9-empty ( Fig. 7d ). We confirmed some of the most differentially expressed genes within these gene sets ( Irf7 and Itgb6 ) by qRT–PCR ( Fig. 7c ). In summary, Tert treatment can modulate transcriptional programmes that favour survival and regeneration after MI, and that resemble the gene expression signature of the neonatal heart. Here we set out to investigate the potential therapeutic role of telomerase activation during MI, a condition with often fatal outcomes in humans. Telomerase is the key enzyme for maintaining TL, which in turn is a molecular determinant of organismal ageing [8] . In an analogous manner to the loss-of-the-heart full regenerative potential that occurs within the first week of life in mice, telomerase expression is also repressed a week after birth in many mouse tissues [23] , [24] . The absence of active telomerase in most somatic cells leads to progressive telomere shortening, eventually leading to age-related diseases, including cardiac dysfunction both in mice and humans [8] , [19] , [20] , [21] . Re-expression of the catalytic subunit of telomerase, Tert , in a Tert -null mouse model is sufficient to reverse premature ageing phenotypes in these mice [46] , and, most interestingly, can also delay physiological ageing in WT mice [27] . Although expression of Tert has been proposed to have non-telomeric functions, which are independent of its catalytic activity [28] , we recently demonstrated that the anti-ageing effects of telomerase require catalytically active Tert [27] . Based on these observations, here we hypothesized that WT Tert expression in the adult heart may have a protective effect from MI by aiding regeneration. Indeed, an increase of Tert -expressing cells has been recently reported in the injury zone and its vicinity after cryoinjury of the heart (an alternative to LAD ligation to induce damage), supporting a role for Tert in infarct healing [47] . The findings described here indicate that WT Tert expression specifically targeted to the heart improves heart functional parameters, decreases scar formation, increases tissue remodelling and potentially regeneration, as well as increases mouse survival after MI. These beneficial effects are coincidental with a net increase in TL in cardiomyocytes 9 weeks post infection. In particular, Tert treatment resulted in improved ventricular function as determined by echocardiography and in a higher metabolic activity in the LV as determined in PET scan analysis. Moreover, Tert treatment resulted in lower rates of fibrosis as indicated by smaller scar sizes in the infarct zone and less interstitial fibrosis in the infarct remote myocardium. Thus, lower deposition of ECM and therefore lower stiffness of the non-infarcted ventricle may in turn explain the 17% increased survival of the Tert -treated mice as well as their higher resistance to external stresses such as the PET procedure. At the molecular level, Tert treatment significantly decreased ANP levels. ANP is part of a fetal gene expression programme, which in humans is one of the first detectable molecular changes during the development of cardiac hypertrophy [2] . Interestingly, the cardiac protective traits of β-blockers are partially attributed to a reversal of fetal gene expression including ANP repression [48] , suggesting a cardio protective role for Tert . Serum metabolite profiling and gene expression analysis on MI revealed elevated EGF serum levels in the Tert -treated mice compared with those treated with empty virus. Signalling via the EGF receptor is known to provide cardio-protection in vivo under conditions of chronic heart failure [41] , again highlighting a cardio protective effect of Tert . Tert treatment also resulted in upregulation of pathways involved in ECM remodelling (increased MMP-9 serum levels and TGF-β signalling). TGF-β exerts pleiotropic effects on virtually all cell types implicated in myocardiac injury, repair and remodelling [49] . Although upregulation of these pathways may seem contradictory given the lower rates of fibrosis and less severe infarcts in the Tert -treated group, prolonged activation of remodelling genes might be also a consequence of increased heart regeneration and this would require sustained ECM remodelling to integrate new cardiomyocytes into the heart matrix. Indeed, cardiomyocytes can re-enter cell cycle after cardiac damage [50] , [51] . In line with this, we found increased numbers of cycling cardiomyocytes in the infarct vicinity in the Tert -treated group. It is therefore tempting to speculate that Tert expression may aid regeneration. However, ultimate demonstration that cardiomyocyte proliferation is stimulated by telomerase expression and the extent to what this contributes to functional heart recovery following MI warrants further investigation using genetic models to trace cardiomyocyte proliferation and cardiac regeneration [52] . In this regard, even though we find higher numbers of cycling cardiomyocytes both by Ki67 and H3 stainings, we cannot rule out that other processes such as cardiomyocyte preservation or after the ischaemic event may also contribute to the better overall heart condition in Tert -treated animals. In addition, our study falls short to explain the origin of the newly formed cardiomyocytes. In this context, their origin has remained obscure and several scenarios had been proposed, including multipotent stem cells, unipotent progenitors, pre-existing differentiated cells, transdifferentiation of cell of other origin or dedifferentiation of cardiomyocytes that re-enter the cell cycle [54] . However, a very recent seminal study convincingly demonstrated that the dominant source of new cardiomyocytes is pre-existing cardiomyocytes and that cardiac injury stimulates their division [53] . Interestingly, pre-existing cardiomyocytes are also the source of newly formed cardiomyocytes in neonatal mice and lower vertebrates such as the zebrafish [6] , [55] . GSEA analysis also identified overexpression of Timp1 , Thbs1 and Thbs4 in the Tert -treated group. These genes are important for cardiac adaptation after MI. TIMP-1 is an anti-apoptotic and anti-fibrotic protein and its overexpression decreases scar size and interstitial fibrosis concomitant with improved cardiac function parameters in the setting of embryonic stem cell therapy after MI in mice [56] . Thbs1 has been suggested to play an important role in the suppression inflammatory responses through TGF-β activation [45] , and therefore may prevent expansion of fibrous remodelling from the infarct zone into the non-infarcted heart. Thbs4 is also an important regulator of cardiac fibrosis and remodelling, whose deletion results in excessive deposition of ECM proteins [43] . Thus, overexpression of Timp1 , Thbs1 and Thbs4 in Tert -treated animals may contribute to its effects in reducing fibrosis, downregulation of inflammatory pathways and overall improved cardiac functions and survival. Finally, we compared our Tert gene expression data with the expression profiles in hearts of neonatal mice (day 1) when cardiomyocytes are highly proliferative. Mice undergo profound transcriptional changes within the first days of life, which coincide with cell cycle exit of cardiomyocytes and the loss of the heart’s regenerative potential [7] . Strikingly, we found that genes associated with increased regenerative capacity (overexpressed at day 1) are significantly enriched in Tert -treated animals. Conversely, genes downregulated in neonates are underrepresented in AAV9- Tert compared with AAV9-empty. Thus, Tert treatment causes a gene expression bias towards a regenerative and proliferative signature found in neonatal mice that are able to fully recover after MI [6] , [7] , which agrees with the suggested increase in cycling cardiomyocytes. Finally, we found increased Tert mRNA levels up to 6 weeks after MI (experimental endpoint), in agreement with stable long-term expression of these vectors [27] , thus suggesting that the beneficial effects of Tert in the regenerative and proliferative potential of the myocardium can be sustained in time by using this strategy. In summary, the findings presented here demonstrate that telomerase activation in the adult heart is beneficial for survival in the murine model after acute MI, which is coincidental with longer telomeres and activation of several pathways associated with cardiac protection and regeneration. These findings serve as proof of concept for the development of innovative strategies based on telomerase activation to treat chronic and acute heart failure. Mice and animal procedures WT mice of pure FVB/N background were used for LAD ligation procedures. Tert heterozygous mice generated as previously described [57] were backcrossed to >98% C57/BL6 background. Tert +/− mice were intercrossed to generate first generation (G1) homozygous Tert −/− knockout mice. All mice of a FVB/N and C57/BL6 background were produced and housed at the specific pathogen-free barrier area of the CNIO, Madrid. All animal procedures were approved by the CNIO-ISCIII Ethics Committee for Research and Animal Welfare (CEIyBA) and conducted in accordance to the recommendations of the Federation of European Laboratory Animal Science Associations. After weaning, five mice were housed per cage and fed ad libitum of a non-purified diet (no. 2018, Harlan). MI was induced in 1-year-old male mice by permanent LAD coronary artery ligation under isofluorane anaesthesia. The analgesic bupenorphine was administered via intraperitoneal injections before the procedure. A sham operation was performed in control and injected mice (see Supplementary Fig. 2 ). Sham operation consists of the same surgery procedure, except from ligation of the LAD. Surgery was performed by a trained animal technician who had no knowledge of the virus treatment to assure randomization of the mouse cohorts. The date of euthanasia was used to estimate mouse survival. For an assessment of post MI survival, mice were followed and inspected daily up to 6 weeks after LAD ligation. Viral particle production Viral vectors were generated as described by Matsushita et al . [58] and purified as previously described [59] . Briefly, vectors were produced through triple transfection of HEK293T. Cells were grown in roller bottles (Corning, NY, USA) in DMEM medium supplemented with fetal bovine serum (10% v/v) to 80% confluence and then co-transfected with the following plasmids: plasmid_1 carrying the expression cassette for gene of interest flanked by the AAV2 viral ITRs; plasmid_2 carrying the AAV rep2 and cap9 genes; plasmid_3 carrying the adenovirus helper functions (plasmids were kindly provided by K.A. High, Children’s Hospital of Philadelphia). The expression cassettes were under the control of the cytomegalovirus (CMV) promoter and contained a SV40 polyA signal for EGFP and the CMV promoter and the 3′-untranslated region of the Tert gene as polyA signal for Tert . AAV9 particles were purified following an optimized method using two caesium chloride gradients, dialysed against PBS, filtered and stored at −80 °C until use [59] . Viral genome particle titres were determined by a standardized quantitative real-time PCR method [60] and primers specific for the CMV sequence (see Supplementary Table 4 ). Virus transduction efficiency and working concentration To assess viral tropism, a control groups of mice (three per virus concentration) were injected with different concentrations of AAV9-CMV- EGFP or AAV9- Tert (1,2 and 5 × 10 11 viral genomes per mouse and 1 × 10 12 viral genomes per mouse) in 100 ul PBS via tail vein injection. At 4 weeks post-injection mice were killed and subjected to either pathological analysis or eGFP and Tert expression assessments. Quantification of eGFP immunostainings was determined by counting the number of peroxidase-stained cells over the total number of haematoxylin-stained cells (liver and brain), or the peroxidase-stained area relative to total section area (heart). Telomerase expression in different tissues was analysed by western blot analysis, qRT–PCR and TRAP (telomerase repeat amplification protocol) assay using whole-cell RNA or protein extracts. To determine viral genome copy number, total DNA was isolated with a MasterPureDNA Purification Kit (Epicentre) from overnight tissue digestions in proteinase K (0.2 mg ml −1 ). The vector genome copy number in 100 ng of total DNA was determined by quantitative PCR with primers and probe specific for the CMV promoter in the AAV vector (see above). The final values were determined by comparison with a reference standard curve built from serial dilutions of the linearized plasmids bearing the CMV-GFP expression cassette spiked into 100 ng of non-transduced genomic DNA. Echocardiography imaging Transthoracic echocardiography was performed with a Vevo 770 high-resolution small animal system (Visualsonics, Canada), the scan probe was RMV707b, with a 40-Mhz frequency, specific for mice ultrasounds. The frame rate was 100 Hz and FOV (field of view) 11 × 11 mm. Animals were anaesthetized with Isofluorane (Isovet, Braun Vetcare), with a 4% during anaesthetic induction and 2% as maintenance level. The analysis was performed placing the ROI (region of interest) over the LV in systole and diastole following the procedure described by Gao et al . [34] Micro PET imaging Images were acquired using eXplore Vista PET-CT (GE Healthcare). Mice were injected with 15 MBq of 18F-FDG (ITP Cyclotron, Madrid) into the lateral tail vein in a volume of 0.1 cc. During imaging, mice were anaesthetized with a continuous flow of 1% to 3% isoflurane/oxygen mixture (2 l min −1 ) 45 min after radiotracer injection. MicroPET scans were performed at 20 min per bed, only one bed per mice placed into the cardiac area. PET images were reconstructed with three-dimensional Ordered Subsets Expectation-Maximization (OSEM) reconstruction and were analysed using MMWS software (eXplore Vista, GEHC) [61] . Histology Hearts were fixed in phosphate-buffered 4% formaldehyde, embedded in paraffin and sectioned (2 mm in thickness) from basal, midventricular and apical regions using a heart slicer (Zivic Instruments, HSMS001-1). Hearts slide sections (5 μm) were stained with Masson’s trichrome. Infarct size and fibrotic length were calculated as the average ratio of scar length to total LV circumference of mid-ventricular sections. Interstitial fibrotic area was performed on Masson’s trichrome-stained transverse heart sections in a semi-quantitative way using the ImageJ software. Three images per heart from the infarct remote area were analysed. Heart morphometric measurements were done on Periodic acid–Schiff-stained midventricular transversal heart section. Measurements taken (distances in μm) were as follows: LVT=left ventricle wall thickness, LV=left ventricle, IVST=interventricular wall thickness, RV=right ventricle, RVT=right ventricle wall thickness and CMCSA=cardiomyocyte cross sectional area; measurements were done using the Panoramic Viewer software. Left ventricular mass (LVM) was calculated as: LVM ( g )=1.04 ([LVT+LV+IVST] 3 −[LV] 3 )−14. LVM index was calculated as: LVMA=LVM/BSA (body surface area). Individual cardiomyocyte size was measured from cells with central nucleus, in the vicinity of infarct areas with clear cell boundaries. A minimum of 20 cardiomyocytes per section was assessed. Immunohistochemistry and immunofluorescence was performed on deparaffinized tissues sections and processed with the indicated antibodies and concentrations: rabbit anti-EGFP, 1:200 (Abcam, ab290); mouse anti EGFP, 1:100 (Roche); rabbit anti-Vimentin, 1:100 (D21H3; Cell Signaling, 5741); mouse anti-heavy chain cardiac Myosin, 1:50 (Abcam, ab15); mouse anti-Troponin T, 1:50 (Thermo Scientific, Ab-1); rabbit anti-KI67, 1:200 (Abcam, ab16667); rabbit anti-active caspase 3, 1:500 (Abcam, ab13847); rabbit anti-phospho-Histon H3, 1:200 (Millipore, 06-570). Quantitative real-time PCR and western blottings Total RNA from tissues was extracted with Qiagen’s RNeasy mini kit, according to the manufacturer’s instructions. Before processing, RNA samples were DNaseI treated. Quantitative real-time PCR was performed using an ABI PRISM 7700 (Applied Biosystems). Primer used in this study are listed in Supplementary Table 4 . Statistical analyses (Student’s t -test) were performed on ΔΔ C t values. Western blottings were made with whole-cell extracts from the indicated tissues with the following antibodies and concentrations: rabbit anti-h/TERT, 1:500 (Calbiochem); rabbit anti-GAPDH, 1:2,000 (Sigma). Quantification was done using the Scion Image Software. For uncropped scans of western blotting, please see Supplementary Fig. 12 . Telomere analysis Q-FISH determination on paraffin-embedded tissue sections was performed as described previously [62] . After deparaffinization, tissues were post fixed in 4% formaldehyde for 5 min, washed 3 × 5 min in PBS and incubated at 37 °C for 15 min in pepsin solution (0.1% Porcine Pepsin, Sigma; 0.01 M HCl, Merck). After another round of washes and fixation as mentioned above, slides were dehydrated in a 70%–90%–100% ethanol series (5 min each). After 10 min of air drying, 30 μl of telomere probe mix (10 mM TrisCl pH 7, 25 mM MgCl 2 , 9 mM citric acid, 82 mM Na 2 HPO 4 , 70% deionized formamide (Sigma), 0.25% blocking reagent (Roche) and 0.5 μg ml −1 Telomeric PNA probe (Panagene)) were added to each slide. A cover slip was added and slides were incubated for 3 min at 85 °C, and for further 2 h at room temperature in a wet chamber in the dark. Slides were washed 2 × 15 min in 10 mM TrisCl pH 7, 0.1% BSA in 70% formamide under vigorous shaking, then 3 × 5 min in TBS 0.08% Tween20, and then incubated in a 4′,6-diamidino-2-phenylindole (DAPI) bath (4 μg ml −1 DAPI (Sigma) in PBS) before mounting samples in Vectashield (VectorTM). Confocal image were acquired as stacks every 0.5 μm for a total of 1.5 μm using a Leica SP5-MP confocal microscope and maximum projections were done with the LAS-AF software. Telomere signal intensity was quantified using Definiens software. HT-qFISH on peripheral blood leukocytes was done according to ref. 63 . Briefly, 120–150 μl blood was extracted from the facial vein 5 weeks after MI. Red blood cells were lysed (Erythrocyte lysis buffer, Qiagen) and 30–90 k leukocytes were plated in duplicate into clear-bottom, black-walled 96-well plates pre-coated for 30 min with 0.001% poly- L -lysine. Plates were incubated at 37 °C for 2 h and fixed with methanol/acetic acid (3:1, v/v) 2 × 10 min and then overnight at −20 °C. Fixative was removed, plates dried for at least 1 h at 37 °C and samples were rehydrated in PBS. Plates were then subjected to a standard Q-FISH protocol (see above) using a telomere-specific PNA-CY3 probe; DAPI was used to stain nuclei. Sixty images per well were captured using the OPERA (Perkin Elmer) High-Content Screening system. TL values were analysed using individual telomere spots (>10,000 telomere spots per sample). The average fluorescence intensities of each sample were converted into kilobase using L5178-R and L5178-S cells as calibration standards, which have stable TLs of 79.7 and 10.2 kb, respectively [64] . Samples were analysed in duplicate, or triplicate in the case of calibration standards. Serum metabolite analysis Blood samples were collected in tubes without any anticoagulant, 6 weeks after MI. Samples were maintained on ice for 20 min and centrifuged for 15 min at 1,300 g . The serum supernatant was frozen and kept at 80 °C until they were analysed to minimize freeze–thaw degradation [65] . Serum urea concentration in mice was determined in an ABX Pentra400 serum analyser (Horiba Medical). In addition, multi-analyte profile serum analysis (see full table of biomarkers analysed in Supplementary Table 1 ) was performed with RodentMap v3.0 (Myriad RBM). Gene expression analysis Total RNA from frozen heart samples was extracted with Qiagen’s RNeasy kit, RNA integrity analysed in a Agilent Bioanalyzer (samples with RNA integrity index <7.8 were discarded) and analysed on Agilent’s Mouse Genome DNA microarray, following the manufacturer’s instructions and ref. 66 . Briefly, differentially expressed genes were obtained by applying linear models using the R limma package [67] (Bioconductor project, http://www.bioconductor.org ). To account for testing of multiple hypotheses, the estimated significance level ( P -value) was adjusted using the Benjamini and Hochberg false discovery rate (FDR) correction. Those genes with FDR<0.15 were selected as differentially expressed between Tert , empty virus-injected hearts and sham-operated controls. GSEA was applied using annotations from Reactome and Kyoto Encyclopedia of Genes and Genomes. Genes were ranked based on limma-moderated t statistic. After Kolmogorov–Smirnoff testing, those gene sets showing FDR<0.1 (ref. 68 ) were considered enriched between classes under comparison. Statistical analysis A log-rank test was used to calculate the statistical differences in the survival curves of the different mice cohorts. An unpaired Student’s t -test was used to calculate statistical significance of mRNA and protein expression levels, TRAP, heart functional parameters, scar size and interstitial fibrosis. Mann–Whitney U -test was used for serum parameters. Pathological assessment either through heart observation after Masson’s trichrome staining or FDG-PET scans were calculated with the χ 2 -test. How to cite this article: Bär, C. et al . Telomerase expression confers cardioprotection in the adult mouse heart after acute myocardial infarction. Nat. Commun. 5:5863 doi: 10.1038/ncomms6863 (2014). Accession codes: Microarray data have been deposited in the GEO repository under accession code GSE62973 ( http://www.ncbi.nlm.nih.gov/geo/query/acc.cgi?acc=GSE62973 )